Short-time movement ofE. colichromosomal loci depends on coordinate and subcellular localization In bacteria, chromosomal architecture shows strong spatial and temporal organization, and regulates key cellular functions, such as transcription. Tracking the motion of chromosomal loci at short timescales provides information related to both the physical state of the nucleo–protein complex and its local environment, independent of large-scale motions related to genome segregation. Here we investigate the short-time (0.1–10 s) dynamics of fluorescently labelled chromosomal loci in Escherichia coli at different growth rates. At these timescales, we observe for the first time a dependence of the loci’s apparent diffusion on both their subcellular localization and chromosomal coordinate, and we provide evidence that the properties of the chromosome are similar in the tested growth conditions. Our results indicate that either non-equilibrium fluctuations due to enzyme activity or the organization of the genome as a polymer–protein complex vary as a function of the distance from the origin of replication. The classic picture of the bacterial chromosome as a disordered medium [1] , [2] is now recognized as inadequate. The last decade has provided ample evidence [3] , [4] that the ‘nucleoid’, that is, the complex composed of genomic DNA, RNA and associated proteins is highly organized in its dynamics and structure. Chromosome dynamics and organization are intricately entangled with the fundamental physiological processes of genome replication and gene expression, and thus with growth, response to stimuli and ultimately fitness. Understanding the bacterial chromosome is thus a (difficult) open challenge, related to fundamental biology and also to biotechnology and health. Addressing this problem with cell biology techniques was initially difficult because of bacteria-specific challenges (for example, small size) and a general underdevelopment of a field caused by the old paradigm of bacteria as a mere well-mixed chemical reactor [5] . Today, techniques such as fluorescent repressor operator systems [6] and the ParB–GFP fusions parS sequences [7] allow visualization of the location in the cell of specific chromosomal loci to investigate chromosome positioning and dynamics. Some studies of the bacterial chromosome [3] have focussed on the organizational properties valid at particular times, for example, by taking the statistics of the subcellular positioning of loci within a population [8] , [9] , [10] , [11] , [12] , [13] . Other studies measure more directly the variation in time of chromosomal organization, which is fundamentally interconnected with chromosome replication and segregation. The relevant timescales to capture these aspects range from approximately 1 min to 1 h (refs 3 , 14 , 15 ). A major success of these studies is the discovery of a dynamic basis for the so-called ‘macrodomains’ [16] . These are regions spanning roughly one-sixth of the Escherichia coli genome, first evidenced by genetic screening of recombination frequency [17] , and are seen to correlate with the long-time dynamics of chromosomal loci [16] . More recent work showed that chromosome segregation is coordinated with cell division in E. coli by interaction of the protein MatP with the divisome [18] . In another study, Joshi et al. [19] have observed that segregation sometimes proceeds through ‘snaps’, suggesting the existence of energetic or entropic barriers preventing segregation, possibly counterbalanced by active processes such as replication itself. In parallel, a series of interesting studies by Weber et al. [20] , [21] , [22] have addressed the s hort-time (1–100 s, that is, much less than a cell cycle) dynamics of loci, using statistics from tens of thousands measured tracks. The motion of chromosomal loci can be quantified by the amplitude and more generally the functional dependence of their mean square displacement, MSD( t ), where t is the observation timescale (or lag time): In complex fluids, this function is very often a power law in time over several orders of magnitude; the power law exponent is an indication of the underlying structure and dynamical processes [23] . The average in equation (1) is either: (a) a time average over the initial times t 0 , or (b) an ensemble average including many loci tracks, or (c) both, which we will term ‘sliding’ averages, as they involve a moving average along the time intervals of the track. The viscoelastic nature of the bacterial cytosol, and the role of the nucleoid in establishing it are not well characterized [4] . Analysing the thermal motion of tracers embedded within viscoelastic materials is a standard technique in soft-matter physics for extracting material properties [24] , [25] and for information on its underlying structure (for example, the crosslinking architecture of cytoskeletal polymer networks [26] ). Thus, the short-time dynamics of a fluorescent locus contains information about the architecture of its surroundings. At small timescales, the contribution of the dynamics of segregation is negligible, and the observed loci motions should relate more simply to the basic ‘polymer solution’ properties of the chromosome [4] . This idea is supported by the following estimate. Suppose, for example, that the loci segregation dynamics would move a locus by half a cell, about 1–3 μm, in a cell cycle, which is no less than 20 min for the fastest growth conditions. This ‘ballistic’ drift motion, in 10 s, would give a contribution to the MSD of about 10 −4 μm 2 , much smaller than the smallest displacements measured experimentally. The studies of Weber et al. yielded three interesting results. First, individual loci ‘subdiffuse’, that is, explore space slower than Brownian motion, as reflected by a power law scaling of MSD with time with an exponent <1. This behaviour appears to be universal, in the sense that it has been observed for different loci of both E. coli and Caulobacter , and with different drug treatments [20] , and the value cannot be explained by simple polymer models [4] , [27] . The authors surmised that this kind of motion could depend on viscoelastic properties of the surrounding cytosol. Second, the mobility of loci changes when drugs such as antibiotics are applied to the bacteria. Third, the local noise felt by tracked loci, in addition to thermal fluctuations, might also be driven by ‘active’ random forces, produced by enzymes and processive motors (such as polymerases and topoisomerases) [21] . In this study, we look for evidence of differences in the short-time (0.1–10 s) motion of different loci along the chromosome, using high-resolution tracking and a large number of measurements. We investigate the loci motion taking place on timescales even shorter than those explored by Weber et al. , down to the limits of positional resolution. We find a dependence (which is robust to changes in growth conditions) of the motion on the chromosomal coordinate, with the Ter region fluctuating significantly less than other regions. We confirm that the motility of the loci is subdiffusive, but we highlight that there are large variations from locus to locus and some variations with timescales. Last, there are also systematic differences of the short-time motility with loci subcellular localization. 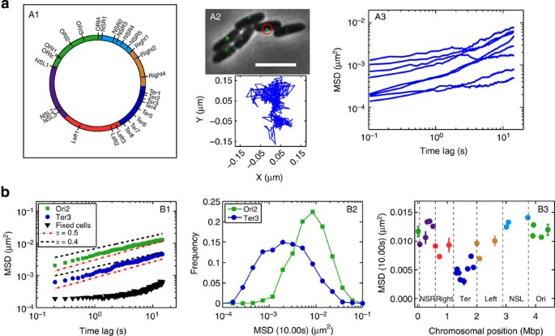Figure 1: Illustration of the experiment and basic results. (a) Pipeline of the analysis. Left (A1): scheme of the loci analysed in this work, arranged around the chromosomal coordinates. The different coloured sectors are the macrodomains and non-structured regions (NSR, NSL) defined in ref.17. The origin of replication is next to the OriC locus (Supplementary Table S1). Middle (A2): illustration of the experiment. The top panel is an overlay of fluorescence and phase contrast pictures (scale bar, 5 μm) ofE. colibacteria growing in agar (minimal medium supplemented with casamino acid and glucose, cell cycle time 75 min, seeSupplementary Methods) with nine visible fluorescently labelled Ter3 loci. The bottom panel shows the tracked movement of the circled fluorescent dot (433 frames long, there are 0.104 s between frames). Right (A3): time-averaged single-track MSD extracted from the nine tracks shown in the middle panel. (b) The short-time displacement of chromosomal loci varies with chromosomal coordinate. Left (B1): plot of the ensemble-average MSDs as a function of time lag, for 1749 tracks of Ori2locus and 974 tracks of Ter3locus (in M9 medium supplemented with casamino acid (CAA) and glucose). As a reference of the background, we show averages from fixed cells. Lines are reference power laws with the annotated exponents. Middle (B2): histogram of MSD at a lag time of 10 s for the same loci shown in the left panel (the curves are colour coded as in the left panel). Right (B3): MSD at a 10-s lag time for all the considered loci inM9 minimal medium supplemented with CAA and glucose. Error bars (s.d.) are computed on at least three different biological realizations (where given). Precision measurement of single loci tracks Figure 1a illustrates the experimental tracking procedure, developed from refs 28 , 29 (see Supplementary Methods and Supplementary Fig. S1 ). Example plots of MSD as a function of time lag from a few loci belonging to a single movie of clonal cells are shown in Fig. 1a . In total, we measured about 150,000 tracks from 156 experiments ( Supplementary Table S1 ). It should be pointed out that, as in previous studies [20] , [21] , these data yield no information on the stage of the cell cycle where a track was taken. As we will see, cell-cycle variability contributes to variance in the data, which have to be regarded as cell-cycle averages. To overcome this limitation, for a smaller set of experiments, we controlled for subcellular localization of loci and cell size, which are both cell-cycle related. Figure 1: Illustration of the experiment and basic results. ( a ) Pipeline of the analysis. Left (A1): scheme of the loci analysed in this work, arranged around the chromosomal coordinates. The different coloured sectors are the macrodomains and non-structured regions (NSR, NSL) defined in ref. 17 . The origin of replication is next to the OriC locus ( Supplementary Table S1 ). Middle (A2): illustration of the experiment. The top panel is an overlay of fluorescence and phase contrast pictures (scale bar, 5 μm) of E. coli bacteria growing in agar (minimal medium supplemented with casamino acid and glucose, cell cycle time 75 min, see Supplementary Methods ) with nine visible fluorescently labelled Ter3 loci. The bottom panel shows the tracked movement of the circled fluorescent dot (433 frames long, there are 0.104 s between frames). Right (A3): time-averaged single-track MSD extracted from the nine tracks shown in the middle panel. ( b ) The short-time displacement of chromosomal loci varies with chromosomal coordinate. Left (B1): plot of the ensemble-average MSDs as a function of time lag, for 1749 tracks of Ori2 locus and 974 tracks of Ter3 locus (in M9 medium supplemented with casamino acid (CAA) and glucose). As a reference of the background, we show averages from fixed cells . Lines are reference power laws with the annotated exponents. Middle (B2): histogram of MSD at a lag time of 10 s for the same loci shown in the left panel (the curves are colour coded as in the left panel). Right (B3): MSD at a 10-s lag time for all the considered loci in M 9 minimal medium supplemented with CAA and glucose. Error bars (s.d.) are computed on at least three different biological realizations (where given). Full size image The MSD calculated from single tracks can be analysed separately ( Fig. 1a ), or data from different tracks can be used to produce ensemble-averaged MSD (that is, the average over an ensemble of ‘random walkers’ following the experimental tracks from the same initial position), as plotted in Fig. 1b . The ensemble-averaged MSD is obtained by fixing t 0 as the time corresponding to the first image of a track. As a measure of background, one can consider the MSD of loci from fixed cells at the same time lag t . Figure 1b also shows the distribution of MSD (10 s) (averaged over t 0 ) for two example chromosomal loci, Ori2 and Ter3. Loci displacement varies with chromosomal coordinate Figure 1b also shows that the distances travelled by loci with different chromosomal coordinate are not the same. For example, the Ori2 and Ter3 loci have large differences in their displacement. Their ensemble-averaged mean square displacement curves are separated by at least a factor of four. The distributions of MSD (10 s) are overlapping, but clearly separated. This trend is the most important finding of this work. Although it is known [16] that the displacements of loci belonging to different macrodomains are different at long timescales (>1 min), these are the first experiments addressing this point at short timescales. This is relevant, as at the timescales of 0.1–10 s the measurement of displacement is a more direct probe of the chromosome physical organization and its noise properties, and is free from the contribution of larger time- and length-scale chromosome rearrangements, such as chromosome segregation dynamics. Previous studies of loci tracking, exploring down to a time resolution of 1 s with high statistics, did not address or report any differences in mobility with chromosomal coordinate [20] , [21] . Contrary to the measurements performed at long lag times [16] , where macrodomains are sharply defined, we find a ‘smoother’ chromosomal trend; Fig. 1b shows the data for the MSD at a 10-s lag time, as a function of the chromosomal coordinate, varying approximately linearly from Ori to Ter for all the considered loci. As discussed above, the Ter proximal loci have an MSD almost an order of magnitude lower than the Ori proximate loci. The trends are robust to growth conditions ( Supplementary Fig. S2 ). We also performed loci tracking in a microfluidic chemostat with finer control over growth conditions [30] and obtained the same results ( Supplementary Fig. S3 ). Given the large statistics considered, the s.e.m. is very small (comparable to symbol size in Fig. 1b ), while the actual spread in the data can be considerable ( Fig. 1b ). Although the observed smooth trend of typical displacement with chromosomal coordinate is consistent with the existence of macrodomains, it would not in itself allow the definition of chromosomal macrodomain boundaries. Heterogeneous subdiffusive exponents from single tracks In agreement with previous studies [20] , we generally find loci exponents following power laws MSD( t )~ t α , very clearly subdiffusive (compatible with exponents α ≤0.5 and often close to α =0.4, see Fig. 1b , Supplementary Note 1 , and Supplementary Figs S4 and S5 ). The analysis of single time-averaged tracks is complementary to the results discussed above. Power law fits of individual MSD( t ) plots give histograms ( Fig. 2 ) of exponents that are in general very wide. The overall histogram ( Fig. 2a ), obtained from all (63540) tracks of a single growth condition, is compatible with previously published results: there is a wide distribution for α (ref. 20 ), which can be rationalized as a finite-size effect of limited length loci tracks (see ref. 27 ). The mean exponent agrees with that of the ensemble averages. Notably, the same histograms plotted for tracks from single loci have similar properties ( Fig. 2a and b ), which was not reported previously. 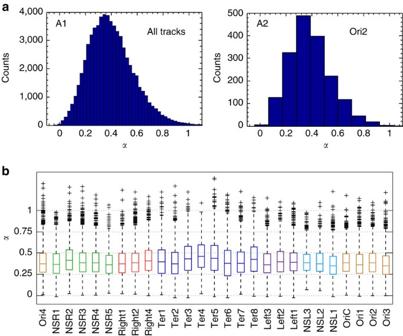Figure 2: MSD exponents of individual tracks. The exponents are fitted in the interval of lag times 0.42–10.09 s and have a wide distribution, which is typically peaked around the exponent valueα=0.4. The data refer to cells grown in M9 minimal medium supplemented with casamino acid and glucose. (a)α-Exponent distribution for all tracks of all loci (63,540 data points) in this condition (A1) and distribution of MSD exponentαfor 1761 individual tracks for the Ori2 locus (A2). (b) Boxplot representation of theαexponent histograms for all individual loci. All medians are around 0.4, with the exception of the Ter macrodomain loci, which appear to have slightly higher median exponents. Figure 2b shows that for all loci, the median exponent α of single tracks is close to 0.4, with a few loci, mostly within the Ter macrodomain, having slightly higher median values and wider distributions. Figure 2: MSD exponents of individual tracks. The exponents are fitted in the interval of lag times 0.42–10.09 s and have a wide distribution, which is typically peaked around the exponent value α =0.4. The data refer to cells grown in M9 minimal medium supplemented with casamino acid and glucose. ( a ) α -Exponent distribution for all tracks of all loci (63,540 data points) in this condition (A1) and distribution of MSD exponent α for 1761 individual tracks for the Ori2 locus (A2). ( b ) Boxplot representation of the α exponent histograms for all individual loci. All medians are around 0.4, with the exception of the Ter macrodomain loci, which appear to have slightly higher median exponents. Full size image To gain further insight into these measurements, we simulated fractional Brownian motion with different exponents (using the algorithm of Deng et al . [31] ). We analysed the simulated distributions and checked if the exponent 0.4 (which points to non-trivial physical organization [4] , [27] ) could be distinguished from 0.5, which corresponds to more conventional ‘Rouse’ subdiffusion of polymer solutions [32] . Comparison of the ensemble-averaged MSD and the single-track α exponent histograms from experiment and simulation ( Supplementary Fig. S6 ) indicates that: (i) the histogram of the simulated data is not as wide as the ones measured experimentally, and (ii) the ensemble-averaged MSD( t ) plots should allow us to discern the exponent from the experimental data. Apparent diffusion varies with chromosomal location Beyond the exponent α , our main focus here is the displacement of a locus at a given (short) timescale, for which we have observed a previously unreported variation along the chromosomal coordinate ( Fig. 1b ). We ask here whether this behaviour is robust over different observation timescales. The subdiffusive behaviour of a probe is generally characterized by the prefactor, through the law MSD( t )=4 D app t α , where D app is called the ‘apparent diffusion constant’. A consistent definition of D app requires that the measured displacements are coherent over different timescales. Thus, we asked whether a collective rescaling of MSD for all loci, assuming the single-exponent value α ≈0.4, would give an acceptable collapse along the whole chromosomal coordinate, despite of the diversity found in the exponents. This procedure proves rather effective. 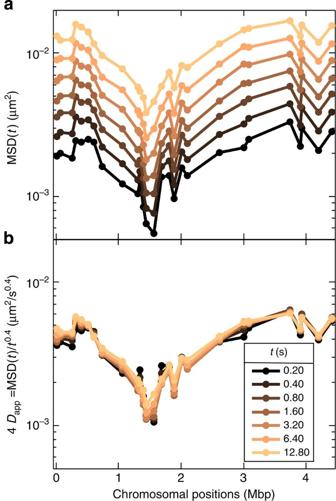Figure 3: Definition of the apparent diffusion constant over different timescales. (a) MSD for all loci shown as a function of chromosomal coordinate (log scale for theyaxis). Different curves refer to different time lagsτ, each separated by a factor of two. The fact that the curves are roughly equally spaced indicates coherence over the range of timescales. (b) A mean apparent diffusion constantDappcan be defined robustly over different timescales. Collapse of the curves shown in the left panel assuming an exponentα=0.4. This operation defines coherently an apparent diffusion constantDapp, which varies with chromosomal coordinate. Figure 3 shows that the mean apparent diffusion constant D app can be defined robustly, because the MSD over different timescales collapses very well onto a single curve by assuming α =0.4. This is a further confirmation and consistency check of the main result of this work: the subdiffusive mobility of loci varies with chromosomal coordinate. Discrepancies with respect to this robust collapse of loci displacements are found in two cases: at short timescales (darker symbols in Fig. 3 ) across the whole chromosome, and for Ter proximal (low mobility) loci. This is simply a mirror of the discrepancies observed in evaluating the exponents and indicates that, despite the coherence between the data, not all loci and timescales perfectly match the single-exponent behaviour (due to experimental errors, physical processes, or both). Figure 3: Definition of the apparent diffusion constant over different timescales. ( a ) MSD for all loci shown as a function of chromosomal coordinate (log scale for the y axis). Different curves refer to different time lags τ , each separated by a factor of two. The fact that the curves are roughly equally spaced indicates coherence over the range of timescales. ( b ) A mean apparent diffusion constant D app can be defined robustly over different timescales. Collapse of the curves shown in the left panel assuming an exponent α =0.4. This operation defines coherently an apparent diffusion constant D app , which varies with chromosomal coordinate. Full size image Apparent diffusion varies with subcellular localization In general, the loci with the highest track variability belong to the Ter proximal region. It has been reported that the Ter macrodomain is preferentially found near the cell periphery [8] and that it is compacted by the protein MatP (ref. 33 ), and possibly subject to tethering interactions at least in certain parts of the cell cycle [18] . The measurements made here could reveal these features. To gain further insight into this observation, we considered the displacements at fixed time lags as a function of loci subcellular localization. A phase contrast image was recorded before acquiring each movie, and segmented to identify loci localization in cell coordinates ( Fig. 4a ). We did not observe interesting trends along the transverse coordinate, and therefore projected the data onto the main axis; the position of each fluorescent dot is thus represented by a single coordinate x ranging from 0 (mid-cell) to 0.5 (cell poles), and thus normalizing cell length to 1. For each loci type, we measured the distribution of x ( Fig. 4b ). 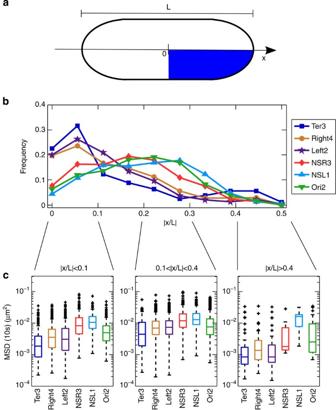Figure 4: Variation of short-time displacement with loci subcellular localization. (a) Sketch of the coordinate system for segmented cells. As the cell orientation is unknown in the experiment, all data are projected onto one cell qurter (shaded area). Data are further projected on the cell long axis to define the coordinatex. (b) Histogram of the density of loci found as a function of long-axis coordinate. One locus per macrodomain is chosen. The Ori2, NSL1 loci are found more often at quarter-cell proximal positions, while the Ter3, Right4 and Left2 loci are found more often close to mid cell. (c) Boxplots of single-track MSD distributions at a time lag of 10 s for the chosen loci for three main coordinate bins, corresponding to mid cell quarter-cell and the cell poles. The short-time apparent diffusion of the Ter3, Right4 and Left2 loci increase when they are found at quarter-cell proximal position (middle panel) compared with cell-pole or mid-cell (left and right panel). This trend is absent or less marked for the other probed loci. Data refer to M9 minimal medium with glucose and casamino acid. Figure 4: Variation of short-time displacement with loci subcellular localization. ( a ) Sketch of the coordinate system for segmented cells. As the cell orientation is unknown in the experiment, all data are projected onto one cell qurter (shaded area). Data are further projected on the cell long axis to define the coordinate x . ( b ) Histogram of the density of loci found as a function of long-axis coordinate. One locus per macrodomain is chosen. The Ori2, NSL1 loci are found more often at quarter-cell proximal positions, while the Ter3, Right4 and Left2 loci are found more often close to mid cell. ( c ) Boxplots of single-track MSD distributions at a time lag of 10 s for the chosen loci for three main coordinate bins, corresponding to mid cell quarter-cell and the cell poles. The short-time apparent diffusion of the Ter3, Right4 and Left2 loci increase when they are found at quarter-cell proximal position (middle panel) compared with cell-pole or mid-cell (left and right panel). This trend is absent or less marked for the other probed loci. Data refer to M9 minimal medium with glucose and casamino acid. Full size image For this subcellular localization study, we considered one locus from each of the six macrodomain regions (see Supplementary Methods ). The locus within the Ter macrodomain, and to a lesser extent the loci within the right and left macrodomains, are found with a higher probability near mid-cell, consistent with previous findings [16] . It is well known that the Ter macrodomain is found at mid-cell before the cell divides, after which it is located at the daughter cell poles. The Ori and non-structured region loci are more broadly distributed, and slightly depleted from mid-cell and from the poles [3] . The boxplots in Fig. 4c show the mobility at these six chromosomal positions, resolved by subcellular localization. At mid-cell and near the poles, the Ter, right and left macrodomain loci show reduced apparent diffusion. Those same loci, when they are away from mid-cell and the poles, move much more. In fact, their displacement is statistically indistinguishable from that of the non-structured and Ori proximal loci. Thus, there is a strong correlation between the localization of a chromosomal segment and its short-time motion, suggesting differences in the physical organization of the chromosome throughout the cell cycle. As one expects a correlation between late cell cycle behaviour and long cells, we have also considered the variation of the apparent diffusion of the same set of loci with cell length ( Supplementary Fig. S7 ). We found that longer cells had decreased diplacement of Ter3 loci and increased displacements of Left2 loci. The former observation could be rationalized by the condensation of the Ter loci before cell division, and the latter by the localization of Left2 near quarter-cell positions (where we find it to have a higher apparent diffusion) in the same part of the cell cycle. The possible sources of error are discussed in Supplementary Note 1 . Stability of apparent diffusion with growth conditions Locus intensity correlates strongly with the measured displacements of both fluorescent chromosomal loci and fluorescent calibration beads ( Supplementary Fig. S8 ). Moreover, in our experiments, the range of loci intensities can vary substantially with nutrient conditions because GFP expression (and plasmid copy number) vary with growth rate [34] . As the measured MSD includes a contribution from both physical dot displacements and dot intensity (which in turn is subject to statistical variation across tracks and loci, see Supplementary Figs S9 and S10 ), care is required when comparing the MSD of loci from cells grown in different nutrient conditions. For example, Fig. 5 shows the MSD at a lag time of 10 s for the Ter3 and the Ori2 loci in three different growth conditions (doubling times 150, 115 and 75 min), parametrized by the intensity of the fluorescence signal. If we computed an average MSD using the distribution of signal intensities for either loci, we would erroneously conclude that the loci mobility varies with growth rate. However, the data indicate that such a conclusion would be based on an experimental artifact caused by differences in GFP expression, as the MSDs of a given locus in different conditions are similar when their intensities are equal. Thus, we have to conclude that the variation of MSD with tested growth conditions should be considered ‘small’ (at our current resolution, and considering the fact that the cell-cycle stage is not resolved by out data). Conversely, the difference of average MSD between two loci is consistent throughout the available intensity range, and the intensity distributions of different loci at equal growth conditions are indistinguishable. Thus, previous results are robust to the effects of intensity, and, in particular, the chromosomal trend in MSD is not the result of specific biases in dot intensity with loci chromosomal coordinates ( Supplementary Figs S11, S12 and S13 ). 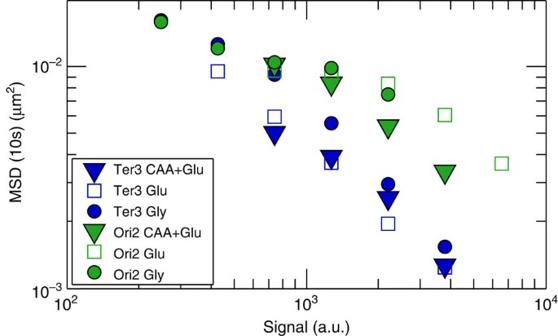Figure 5: Variation of apparent diffusion with growth conditions and dot intensity. The plot shows the mean MSD at a fixed time lag of 10 s for the Ori2 (green) and Ter3 (blue) measured in different growth conditions (represented by different symbols), and parameterized by pixel intensity (xaxis). Circles: minimal medium supplemented with glycerol, doubling time 150 min; squares: minimal medium supplemented with glucose, doubling time 115 min; triangles: minimal medium supplemented with CAAs and glucose, doubling time 75 min. Each point refers to an average performed in a given intensity bin (compare with the calibration plots,Supplementary Fig. S8). As the curves largely overlap where the intensity ranges do, the variation of MSD with growth conditions can be considered small or absent. Conversely, the variation of MSD between the two loci is consistent throughout the available intensity range, and decreases only for the faintest loci. Figure 5: Variation of apparent diffusion with growth conditions and dot intensity. The plot shows the mean MSD at a fixed time lag of 10 s for the Ori2 (green) and Ter3 (blue) measured in different growth conditions (represented by different symbols), and parameterized by pixel intensity ( x axis). Circles: minimal medium supplemented with glycerol, doubling time 150 min; squares: minimal medium supplemented with glucose, doubling time 115 min; triangles: minimal medium supplemented with CAAs and glucose, doubling time 75 min. Each point refers to an average performed in a given intensity bin (compare with the calibration plots, Supplementary Fig. S8 ). As the curves largely overlap where the intensity ranges do, the variation of MSD with growth conditions can be considered small or absent. Conversely, the variation of MSD between the two loci is consistent throughout the available intensity range, and decreases only for the faintest loci. Full size image We performed these measurements with high-precision equipment and techniques, analysing large numbers of tracks, for time lags in the range 0.1–10 s. As we argued, at these timescales the effects of the directed movement associated with the chromosomal segregation ‘choreography’ are negligible. Thus, we believe that our results are not a consequence of segregation dynamics. On the contrary, the properties of loci movement probed here should relate to basic physical properties [4] : the organization and the local non-equilibrium noise of the ensemble formed by the genome and its associated proteins and RNA. Considering a discrete and fast ‘snap’ motion as reported in ref. 19 , one can ask whether this could affect our measurements. We can estimate a snap as a 2-min directed motion relocating a locus by a quarter cell, that is, about 0.25–1 μm. In this case, the apparent MSD (10 s) would be in the range 10 −4 –10 −3 μm 2 , and thus should still be smaller than the detected displacements. Repeating the same estimate for longer time lags, and comparing with our measurements suggests that snap motion could start affecting loci MSD only on timescales around 50–100 s. Obviously, the actual observation of this phenomenon in the statistical averages of loci properties would depend on the typical fraction of cells undergoing snapping motion. Additionally, if the snaps strongly affect the averages, this would likely be visible as a crossover behaviour in the MSD curves. We are currently studying this question in more detail, but the above considerations lead us to exclude that it can affect our results here. We find a dependency of loci short-time subdiffusion on chromosomal location. This happens coherently across different timescales, allowing us to define an apparent diffusion constant D app that varies with loci coordinate. The ‘smooth’ trend of D app is consistent with the existence of macrodomains, but would not allow the definition of their boundaries if they were not known from other experiments [17] . Interestingly, the replichore-symmetric pattern of D app resembles the large-scale binding and transcription patterns related to the action of some nucleoid-associated proteins and topoisomerase [35] , [36] . Previous studies [16] , [17] defined macrodomains as compartments with respect to population-level recombination probability between loci and using dynamic measurements at long timescales (where the stage in the cell cycle is controlled, but the movement of loci could be biased by segregation). Thus, one could imagine that macrodomains might emerge through the segregation dynamics over the cell cycle, and not through the microphysics of the nucleoid. However, it is well known that proteins such as MatP are macrodomain specific [37] , and signatures of macrodomain boundaries appear in various large-scale expression/binding studies [35] , [38] , [39] . Additionally, our data suffer from incomplete control of the cell-cycle stage, and macrodomains might be differentially organized during the cell cycle. Therefore, although it is not possible to draw any definite conclusion, we speculate that both the segregation process and physical transitions of different macrosegments of the genome contribute to the definition of macrodomains at population level. By examining loci dynamics as a function of subcellular position, we found that short-time subdiffusion of loci depends on their subcellular localization. This suggests that local physical properties vary according to specific instants of the cell cycle, which is very plausible to expect, given the observed replication, decatenation, (de)-condensation transitions that the chromosome undergoes over a bacterial cell cycle [34] , [4] , [40] . Notably, this trend is particularly evident for the Ter macrodomain locus, which becomes less mobile at cell poles and at mid-cell, that is, probably around cell division, when the Ter macrodomain is known to be compacted by MatP and possibly externally tethered [16] , [18] , [33] . Conversely, when the Ter macrodomain in its supposed uncompacted state, where it is found all along the cell longitudinal coordinate [8] , [9] , one can expect increased loci motion. We also reported a small variation of (cell-cycle averaged) apparent diffusion with respect to the growth conditions. A recent study by Weber et al. [21] has found that an ATP-dependent term is present in the motion of chromosomal loci. It is important to point out that the two results are not in contrast, as the experiments are performed with different protocols. In the quoted study, the cells are prepared in the same growth conditions, and then exposed to different temperatures before the measurement, while in our case the cells are kept in the same growth medium for a long time and the physiological state is fully adapted. Future studies should move towards (i) analysing the motion in the cell coordinate system and (ii) capturing the cell-cycle dependence. Our results suggest that the subdiffusive nature of chromosomal loci is dictated by stable viscoelastic properties of the ‘complex fluid’ formed by the cytosol and the nucleoid itself, whereas the apparent diffusion constant appears to reflect variation along the chromosome and over the cell cycle. There are two main possible interpretations of these trends, which could also coexist. On the one hand, the local physical organization could vary, for example, differential binding of nucleoid proteins or topoisomerases [35] , [36] could alter the local ‘mesh size’ of the nucleoid, its effective stiffness, and/or the effective hydrodynamic radius of one of its segments. On the other hand, the local noise level could vary, which would allow changes in the local mobility even in an otherwise homogeneous substrate. This is obviously not possible thermally in such an environment, but could be easily realized by active processes [21] , [41] . In other words, differential activity of energy-consuming enzymes could change the amplitude of the fluctuations locally felt by a locus. A non-thermal scaling of D app has been reported by the recent work of Weber et al. [21] , although a precise identification of its source proved to be elusive. The higher apparent diffusion of Ori proximate loci would also be consistent with the higher activity of this region in terms of transcription–translation [42] , and possibly related to the existence of transcription clusters [43] , [44] . Conversely, proteins such as MatP and H-NS bind unevenly on the genome, and give rise to specific clusters [38] , [45] . Furthermore, the combined action of topoisomerases and the HU nucleoid protein forms a very similar genomic pattern to the trend of apparent diffusion constant measured here [35] . Thus, although our data does not allow one to distinguish between the two phenomena, we speculate that they could both be in place. How to cite this article : Javer, A. et al. Short-time movement of E. coli chromosomal loci depends on coordinate and subcellular localization. Nat. Commun. 4:3003 doi: 10.1038/ncomms3003 (2013).